Endonuclease V cleaves at inosines in RNA Endonuclease V orthologues are highly conserved proteins found in all kingdoms of life. While the prokaryotic enzymes are DNA repair proteins for removal of deaminated adenosine (inosine) from the genome, no clear role for the eukaryotic counterparts has hitherto been described. Here we report that human endonuclease V (ENDOV) and also Escherichia coli endonuclease V are highly active ribonucleases specific for inosine in RNA. Inosines are normal residues in certain RNAs introduced by specific deaminases. Adenosine-to-inosine editing is essential for proper function of these transcripts and defects are linked to various human disease. Here we show that human ENDOV cleaves an RNA substrate containing inosine in a position corresponding to a biologically important site for deamination in the Gabra-3 transcript of the GABA A neurotransmitter. Further, human ENDOV specifically incises transfer RNAs with inosine in the wobble position. This previously unknown RNA incision activity may suggest a role for endonuclease V in normal RNA metabolism. RNA editing covalently alter the nucleotide sequence of RNA transcripts relative to that of the encoding DNA, thereby contributing to gene diversity [1] . One of the most prevalent RNA modifications is adenosine (A) deamination, which results in conversion of the 6-aminopurine ring of A to the 6-oxopurine ring of inosine (I) [2] . Inosine has different base pairing properties to A and is interpreted as guanosine (G) in cells. Enzymes catalyzing this conversion are adenosine deaminases acting on RNA (ADARs) [3] , which are conserved enzymes found in most multicellular organisms [4] . Important ADAR targets are mRNAs for neurotransmitter receptors in mammals and editing is critical for normal brain development and behaviour [5] . In all cases, adenosine deamination results in a dramatic alteration of the receptor function [5] . Improper function of ADARs has been correlated with serious neurological and mental human disorders [6] . However, the vast majority of A to I conversions are found in non-coding regions where they are involved in controlling the activity of small RNAs such as short interfering (si)RNA and micro (mi)RNAs [7] , [8] . Inosine is also a central component of transfer RNA (tRNA) where it is found in the wobble position (I 34 ) in the anticodon loop of certain tRNAs [9] . In E. coli , only tRNA Arg (ACG) undergoes A-to-I editing, whereas in eukaryotes seven to eight tRNAs contain I 34 (ref. 10 ). Deamination of A to I is performed by adenosine-specific deaminases acting on tRNA (ADATs), which are homologues of the ADARs. I 34 is crucial for decoding during protein synthesis as wobble I allow for base pairing with C, T and A [9] , [11] . Inosine in ribosomal RNA is unusual [12] . While I is a normal and essential residue in RNA (rI), I in DNA (dI) is regarded as damage because of its miscoding properties. Inosine in DNA is a result of spontaneous or nitrosative stress-induced deamination of dA [13] . To counteract such threats, cells express DNA repair proteins specific for inosine. In E. coli, the primary enzyme for the repair of dI is endonuclease V (EndoV) [14] , which is encoded by the nfi gene [15] . EndoV initiates repair by Mg 2+ -dependent cleavage of the second phosphodiester bond 3′ to the lesion generating 3′-OH and 5′-P termini [14] , [16] , [17] . EndoV incises DNA without removing the inosine nucleotide (nt), thus completion of repair depends on additional proteins, a process that is currently poorly understood. Deaminated adenosines can also be repaired by the base excision repair pathway [18] , [19] . Homologues of EndoV are found in most species, and despite strong sequence conservation robust dI activity has only been demonstrated for the prokaryotic enzymes [20] , [21] , [22] , [23] , [24] , [25] , [26] . Recently, we characterized human ENDOV without detecting any dI incision [21] . Interestingly, when fused to the green fluorescent protein, ENDOV was not found in the nucleus of HeLa cells as expected for a DNA repair protein. Rather, ENDOV localized to nucleoli and the cytoplasm, which are the compartments for RNA. In the present study, we show that human ENDOV has a strong and specific incision activity on RNA substrates containing rI. Also EndoV from E. coli , which is an inosine-specific DNA repair enzyme, cleaves at inosines in RNA. Human ENDOV has a preference for single-stranded substrates, whereas E. coli EndoV is equally active on both single- and double-stranded RNA. These are the novel findings implying a role for endonuclease V in RNA metabolism. Human ENDOV is an inosine-specific ribonuclease ENDOV proteins are highly conserved [16] , a feature that normally reflects conserved function—in this case incision at dI residues in DNA. However, human ENDOV appears to be inactive towards dI [21] . As inosines are not only found in DNA, but are also abundant in RNA, we hypothesized that inosines in RNA could be the substrate for ENDOV. Furthermore, the protein structure of endonuclease V from Thermotoga maritima reveals an ‘RNase H-like motif’ supporting link to RNA [16] . Finally, RNA as a substrate for ENDOV is also consistent with the observation of ENDOV–green fluorescent protein fusion proteins in the cytoplasm and nucleoli of HeLa cells [21] . Therefore, human ENDOV was purified as described and analyzed for activity on single- and double-stranded RNA oligonucleotide substrates with centrally located rI residues ( Supplementary Table S1 ). Interestingly, human, as well as E. coli endonuclease V, efficiently cleaved both the single- (rI) and double-stranded (rI:rU) RNA substrates ( Fig. 1a,b ). Both endonucleases were most effective at the highest pH tested (9.5) when Mg 2+ (5 mM) was used in the reaction, however, with Mn 2+ as the divalent ion, both enzymes were most active at pH 7.5 ( Supplementary Fig. S1a ). At pH 7.5, both enzymes were active over a broad range of Mn 2+ concentrations (0.25–5 mM) ( Supplementary Fig. S1b ). Neither of the enzymes incised an RNA substrate with a cognate rA instead of rI ( Fig. 1c ). Single- and double-stranded DNA substrates with inosine were cleaved by the E. coli enzyme, but not by the human ENDOV ( Fig. 1d,e ) as previously described [21] . 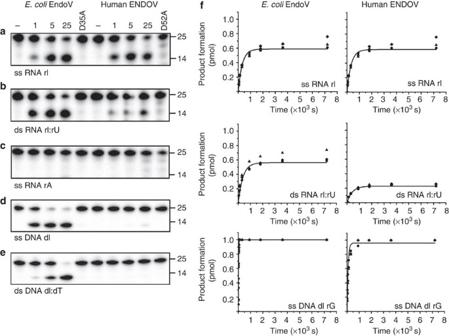Figure 1: Various incision activities forE. coliand human endonuclease V at inosines in DNA and RNA. The substrates (a) single-stranded (ss) RNA rI, (b) double-stranded (ds) RNA rI:rU, (c) ss RNA rA, (d) ssDNA dI, (e) ds DNA dI:dT were incubated with the wild-type enzymes (1–25 nM, as indicated) or the two site-specific mutantsE. coliD35A and human D52A (25 nM) and reaction products analyzed by PAGE. RNA sizes (in nt) are indicated, –=no enzyme added, r=ribonucleotide and d=deoxynucleotide. (f) Single-turnover kinetic analysis with enzyme and substrates as indicated. Figure 1: Various incision activities for E. coli and human endonuclease V at inosines in DNA and RNA. The substrates ( a ) single-stranded (ss) RNA rI, ( b ) double-stranded (ds) RNA rI:rU, ( c ) ss RNA rA, ( d ) ssDNA dI, ( e ) ds DNA dI:dT were incubated with the wild-type enzymes (1–25 nM, as indicated) or the two site-specific mutants E. coli D35A and human D52A (25 nM) and reaction products analyzed by PAGE. RNA sizes (in nt) are indicated, –=no enzyme added, r=ribonucleotide and d=deoxynucleotide. ( f ) Single-turnover kinetic analysis with enzyme and substrates as indicated. Full size image Mapping of the exact position of cleavage revealed that both enzymes nicked the RNA substrate at the second phosphodiester bond 3′ to the deaminated base as expected ( Supplementary Fig. S2a ). Single-turnover kinetic analyses revealed a 1.3-fold higher turnover rate ( k obs ) for human ENDOV on single-stranded than on double-stranded RNA, whereas E. coli EndoV showed the same turnover rate for incision of both the substrates ( Fig. 1f and Supplementary Table S2 ). Inosine-containing DNA appears to be the preferred substrate for E. coli EndoV, as the turnover rate on inosine-containing single-stranded DNA was twice that of single-stranded RNA and five times higher for double-stranded DNA versus double-stranded RNA ( Supplementary Table S2 ). RNAs are transcribed as single-stranded molecules but fold spontaneously under physiological conditions to adopt a secondary structure [27] . Thus, all four combinations of base pairs with rI may form, of which rI:rC is the most stable pair [28] . As double-stranded RNA with a rI:rU pair had already been tested ( Fig. 1b ), the three remaining base pair combinations (rI:rG, rI:rA, rI:rC) were used as substrates in activity assays. E. coli EndoV cleaved all double-stranded RNA substrates with lowest affinity for the rI:rC substrate ( Supplementary Fig. S2b–d ). As is the case for the rI:rU substrate ( Fig. 1b ), human ENDOV also incised the three other double-stranded RNA substrates ( Supplementary Fig. S2b–d ). Site-specific ENDOV mutants were tested for ribonuclease activity. Mutants of the conserved catalytic aspartates ( E. coli : D35A and human: D52A) could not incise the rI substrates ( Fig. 1a–e , Supplementary Fig. S2b–d ). Tyrosine 91 of human ENDOV corresponds to Y80 of T. maritima EndoV, which is a key residue for dI recognition [16] . The ENDOV Y91A mutant displayed wild-type affinity for branched DNA substrates [21] , however, rI incision was totally abolished ( Supplementary Fig. S2e ). The human mutants RK (R248A, K249A) and Wedge (the four residues PYVS[90–93] mutated to four glycines) previously shown to have defective DNA binding [21] were also inactive on RNA ( Supplementary Fig. S2e ). These results confirm that endonuclease V enzymes indeed are inosine-specific enzymes, yet the affinity for DNA versus RNA differs. DNA with a ribonucleotide 3′ to dI is incised by ENDOV Endonuclease V belongs to the same structural family as RNase H enzymes, which specifically cleaves the RNA strand of RNA:DNA hybrids [16] , [29] . RNA:DNA hybrids are formed during DNA replication, RNA transcription and reverse transcription, and adopt a different conformation to double-stranded DNA [30] . To test whether ENDOV has activity for mixed RNA:DNA substrates, two hybrid substrates RNA:DNA- and DNA:RNA-containing rI or dI, respectively, were designed. Human ENDOV cleaved only the hybrid with rI in the RNA strand, whereas E. coli EndoV cleaved both the substrates ( Fig. 2a,b ). From these data, we conclude that human ENDOV cleavage is strictly dependent on ribonucleotides in the inosine containing strand. Specifically, we find that ENDOV is highly active on single-stranded DNA when a single ribonucleotide is present directly following the dI residue ( Fig. 2c ). Hence, the 2′ OH group in this particular ribose seems to be critical and sufficient for incision activity. A model of human ENDOV with rG in this position reveals that the 2′ OH group may interact with the conserved catalytic glutamate (E100) and possibly replace an active site water molecule ( Fig. 2d ). This assumption is based on comparison with the corresponding coordination sphere around Mg 2+ in the active site of T. maritima EndoV in complex with the cleavage product [16] . The difference in activity of human ENDOV between single- and double-stranded DNA with rG next to dI ( Figs 1f and 2c,e ), suggests that the nucleic acid helical structure is also critical for substrate processing; incision activity is only observed for double-stranded inosine substrates having A-form helices, like double-stranded RNA and RNA:DNA hybrids [31] , but not for double-stranded B-form DNA. A B-form DNA may have steric conflicts with surface-exposed residues in human ENDOV. 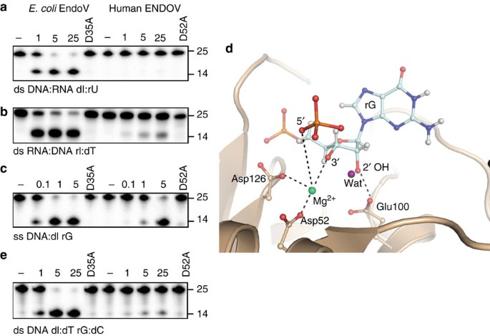Figure 2: Incision activities for human ENDOV on RNA depends on a ribonucleotide 3′ to inosine. The substrates (a) ds DNA:RNA dI:rU, (b) ds RNA:DNA rI:dT, (c) ss DNA dI rG were incubated with the wild-type enzymes (0.1–25 nM, as indicated) or the two site-specific mutantsE. coliD35A and human D52A (25 nM) and reaction products analyzed by PAGE. (d) Structural model of the active site of human ENDOV with a ribonucleotide. The 2′ OH group is close to the conserved glutamate (E100), as well as the active site water molecule (Wat) coordinating the Mg2+cofactor, which bridges the 3′- and 5′-ends in the incised product. (e) The endonuclease V enzymes were tested for activity against the ds DNA dI:dT rG:dC substrate as ina–c). RNA sizes (in nt) are indicated, –=no enzyme added, r=ribonucleotide and d=deoxynucleotide. Figure 2: Incision activities for human ENDOV on RNA depends on a ribonucleotide 3′ to inosine. The substrates ( a ) ds DNA:RNA dI:rU, ( b ) ds RNA:DNA rI:dT, ( c ) ss DNA dI rG were incubated with the wild-type enzymes (0.1–25 nM, as indicated) or the two site-specific mutants E. coli D35A and human D52A (25 nM) and reaction products analyzed by PAGE. ( d ) Structural model of the active site of human ENDOV with a ribonucleotide. The 2′ OH group is close to the conserved glutamate (E100), as well as the active site water molecule (Wat) coordinating the Mg 2+ cofactor, which bridges the 3′- and 5′-ends in the incised product. ( e ) The endonuclease V enzymes were tested for activity against the ds DNA dI:dT rG:dC substrate as in a – c ). RNA sizes (in nt) are indicated, –=no enzyme added, r=ribonucleotide and d=deoxynucleotide. Full size image In vivo and in vivo -like RNAs as substrates for ENDOV The substrates used above are all random oligonucleotide sequences, and to test for activity towards an in vivo deamination target, an oligonucleotide corresponding to a part of the mouse (m)Gabra-3 transcript of the neurotransmitter GABA A was synthesized. This 38 nt RNA has an A in position 27, known to be deaminated by adenosine deaminases ADAR1 and ADAR2, and is referred to as the I/M site [32] . Upon folding of this RNA, rI will form a stable base pair with cytosine (C), whereas an unedited A will form a mismatch with C [32] . Human ENDOV, as well as the E . coli enzyme, generated an incision product of the expected size of 28 nt when assayed with the rI-containing mGabra3 substrate, whereas no activity was seen with the unedited variant ( Fig. 3a,b ). This result suggests that ENDOV could be involved in antagonizing the effect of the ADAR enzymes by destruction of rI-containing transcripts. 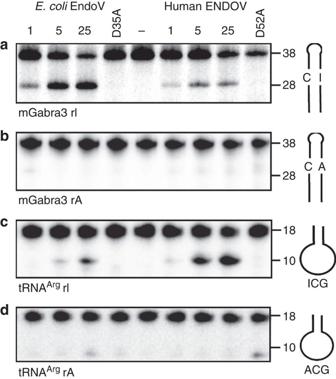Figure 3: Human ENDOV cleaves at inosines inin vivo-like RNA substrates. The substrates (a) mGabra3 rI, (b) mGabra3 rA, (c) tRNAArgrI, (d) tRNAArgrA were incubated with the endonuclease V enzymes (1–25 nM, as indicated) and reaction products analyzed by PAGE. RNA sizes (in nt) are indicated, –=no enzyme added, r=ribonucleotide and glyphs illustrate the different substrates. Figure 3: Human ENDOV cleaves at inosines in in vivo -like RNA substrates. The substrates ( a ) mGabra3 rI, ( b ) mGabra3 rA, ( c ) tRNA Arg rI, ( d ) tRNA Arg rA were incubated with the endonuclease V enzymes (1–25 nM, as indicated) and reaction products analyzed by PAGE. RNA sizes (in nt) are indicated, –=no enzyme added, r=ribonucleotide and glyphs illustrate the different substrates. Full size image Next, a substrate corresponding to the anticodon loop in E. coli tRNA Arg (ACG), wherein the wobble base A34 is the only known A-to-I deaminated tRNA position in prokaryotes [33] , was tested. Cleavage within the anticodon loop of tRNAs is a well-documented response to different stress conditions, such as starvation and oxidation, in different organisms [34] . The rI-containing anticodon substrate, but not the unedited A-containing control substrate, was incised by both enzymes, though most efficiently by human ENDOV ( Fig. 3c,d ). Further, total tRNA isolated from human U373 cells, was incubated with ENDOV and examined for cleavage. Individual tRNAs were detected by Northern blot hybridization using labelled oligonucleotides complementary to the 5′-fragment of the different tRNAs as probes. Full-length processed tRNAs are 71–82 nt long and cleavage next to the wobble A/I would result in products of 35 (5′-fragment) and 36–47 (3′-fragment) nt. Specific cleavage in the anticodon loop of tRNA Ser (AGA), tRNA Leu (AAG) and tRNA Arg (ACG), all known to have rI in the anticodon loop, was demonstrated ( Fig. 4a–c ). In contrast, probes for tRNA Asp (GTC), tRNA Glu (CTC) and tRNA Lys (CTT) lacking A/I 34 editing, revealed no incision products ( Fig. 4d–f ). No general degradation of the tRNA was seen as total tRNA remained intact after incubation with ENDOV ( Supplementary Fig. S2f ). These data could imply a role for ENDOV in fragmentation of tRNAs containing rI. 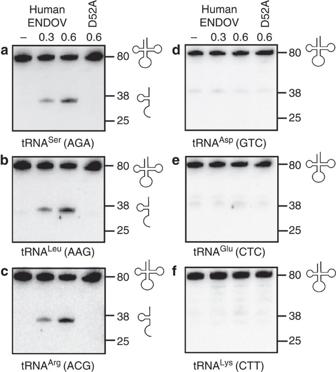Figure 4: Human ENDOV cleaves at inosines in tRNA. Northern blots of tRNA isolated from human U373 cells incubated with human wild-type (0.3 and 0.6 μM) or mutant D52A (0.6 μM) ENDOV enzymes, hybridized with DNA probes complementary to the 5′-termini of (a) tRNASer(AGA), (b) tRNALeu(AAG), (c) tRNAArg(ACG), (d) tRNAAsp(GTC), (e) tRNAGlu(CTC) and (f) tRNALys(CTT). Size markers (80, 38 and 25 nt) are shown and glyphs indicate full-length and fragment tRNA species. Figure 4: Human ENDOV cleaves at inosines in tRNA. Northern blots of tRNA isolated from human U373 cells incubated with human wild-type (0.3 and 0.6 μM) or mutant D52A (0.6 μM) ENDOV enzymes, hybridized with DNA probes complementary to the 5′-termini of ( a ) tRNA Ser (AGA), ( b ) tRNA Leu (AAG), ( c ) tRNA Arg (ACG), ( d ) tRNA Asp (GTC), ( e ) tRNA Glu (CTC) and ( f ) tRNA Lys (CTT). Size markers (80, 38 and 25 nt) are shown and glyphs indicate full-length and fragment tRNA species. Full size image In this report, we demonstrate efficient and specific cleavage at single rI residues in RNA by human ENDOV. ENDOV has activity for both single- and double-stranded RNAs, as well as for edited tRNA anticodon loops containing rI. To our knowledge, ribonuclease activity has not been previously described for endonuclease V, and we propose that ENDOV may have an important role in RNA metabolism. We have previously reported that human ENDOV binds to DNA with higher affinity for branched DNA structures than linear DNA [21] . Here we find that the nucleic acid helical structure is also of importance for ENDOV activity ( Fig. 2c–e ). It appears that the helical conformation (A- or B-form) is more important for binding than the type of nucleic acid (DNA or RNA), whereas catalytic activity is critically dependent on a ribonucletide in the correct position with a 2′ hydroxyl group close to the active site metal cofactor. At present, we do not know whether ENDOV binding to DNA is biologically important or whether it simply reflects a general affinity of ENDOV for nucleic acids. Several reports demonstrate that deamination of adenosine to inosine by the ADAR enzymes has a central function in vivo [5] , [6] . We may speculate that the ribonuclease activity of ENDOV could antagonize the effect of the ADAR enzymes by specific cleavage and destruction of edited transcripts. As many ADAR targets are neurotransmitters, fine-tuning of receptor activity by regulation of the level of edited versus non-edited forms could be of major importance for optimal brain function. It should be mentioned that the Tudor-SN nuclease, which is part of the RISC complex, has also been coupled to cleavage of inosines in RNA [35] , [36] . It is proposed that Tudor-SN cleaves or promotes the cleavage of hyperedited double-stranded RNA by acting as an activator, however, its specific enzymatic properties have not been thoroughly investigated [35] , [36] . Cleavage of tRNAs within the anticodon loop is part of the cellular response to stress conditions such as oxidation and starvation in many organisms [37] . Nucleases responsible for this cleavage have been identified, and defects in tRNA fragmentation are associated with apoptosis, cancer and disease progression [34] . As far as we know, specific cleavage of tRNAs at inosines has not previously been described, but an analogous system is the killer toxin zymocin from Kluyveromyces lactis , which depends on the wobble uridine modification 5-methoxy-carbonyl-methyl for tRNA cleavage [38] . Interestingly, E. coli EndoV was also active on inosines in RNA, demonstrating that EndoV is more than a DNA repair enzyme. Enzymatic deamination of adenosines in RNA appears to be uncommon in prokaryotes, and we may speculate that a more general role exists for endonuclease V enzymes in removal of damaged/deaminated RNA transcripts. Recently, several DNA repair proteins including AlkB/ABH2, SMUG1, APE1 and TDP2 have been shown to possess activity on damaged RNA [39] , [40] , [41] , [42] , [43] and this is suggested to function as a quality control for RNA. In any case, tight regulation of the ENDOV ribonuclease activity to prevent aberrant cleavage, for example, by compartmentalization, post-translational modification or interacting partners, will be of great importance. Expression and purification of endonuclease V enzymes Wild-type and mutants human ENDOV proteins were expressed in E. coli BL21-Codon Plus (DE3)-RIPL cells (Agilent Technologies) as fusion proteins with an N-terminal His-MBP tag [21] . After induction of protein expression with isopropyl β- D -1 thiogalactopyranoside (0.25 mM), bacteria were grown at 18 °C over night. Cells were harvested by centrifugation and the pellet resuspended in 50 mM Tris HCl pH 8.0, 300 mM NaCl, 10 mM imidazole and 10 mM β-mercaptoethanol (β-ME) (buffer A). Cells were lysed by sonication and the cleared lysate applied to Ni-nitrilotriacetic acid affinity chromatography. Recombinant His-MBP-ENDOV was eluted with 300 mM imidazole in buffer A. Peak fractions were pooled and dialyzed at 4 °C in 50 mM Tris HCl pH 8.0, 0.5 mM EDTA, 1 mM dithiothreitol (TEV buffer). TEV protease was added (ratio 1:100) and dialysis continued at 12 °C over night. After proteolysis, the protein mixtures were dialysed against buffer A and the free His-MBP and TEV proteins were separated from ENDOV by a second Ni-NTA purification step. The untagged ENDOV proteins were collected in the flow-through and wash fractions, concentrated and applied to a Superdex 75 size-exclusion chromatography column (GE Healthcare) equilibrated with 50 mM Tris HCl pH 8.0, 50 mM NaCl and 10 mM β-ME. Purified ENDOV was concentrated and stored at −20 °C. The two inactive endonuclease V mutants E. coli D35A and human D52A were made by site-specific mutagenesis using the forward primers 5′-ACCGGATCTGATCGCCGGAGCC GCT GTCGGGTTTGAGCAGGGC-3′ for D35A and 5′-CAGCGTGTGGGCGGTGTG GCT GTTAGTTTCGTGAAAGGTG-3′ for D52A with their corresponding reverse and complementary oligonucleotides (mutated codons are underlined). DNA/RNA substrates All DNA/RNA substrates were oligonucleotides synthesized by The Midland Certified Reagent Company, and are listed in Supplementary Table S1 . The oligonucleotides were 5′-end labelled with [γ- 32 P]ATP (Perkin Elmer) using T4 polynucleotide kinase (New England BioLabs). Polynucleotide kinase was inactivated by the addition of 10 mM EDTA. Double-stranded substrates were made by adding the complementary strand and heating to 55 °C followed by slowly cooling to room temperature. The DNA and RNA substrates were separated by 20% native polyacrylamide gel electrophoresis (PAGE; LongRanger Gel Solution, Lonza, 0.5xTBE), excised from the gel, eluted by diffusion in H 2 O and stored at 4 °C. DNA and RNA incision activities and single-turnover analysis The DNA and RNA nicking assays were performed with 1 nM substrate, 0.1–25 nM of enzyme (as indicated in the figures) and standard reaction buffer (10 mM Tris-HCl pH 7.5, 0.5 mM MnCl 2 , 50 mM KCl, 1 mM dithiothreitol and 5% glycerol) in a total volume of 10 μl or with changes are indicated. To adjust for pH, Tris-HCl, pH 7.5, 8.5 or 9.5 was used and divalent ions kept at 5 mM. When testing Mn 2+ concentrations, Tris-HCl pH 7.5 was used and different amounts of MnCl 2 added (0.25–5 mM). The samples were incubated at 37 °C for 30 min and formamide loading buffer (90% formamide, 0.1% xylene xyanol and 0.1% bromphenol blue) was added to terminate the reactions. Samples were heated to 50 °C for 5 min before separation of substrate and product by 15% denaturating PAGE (Long Ranger, 7 M urea and 1x taurine). To map ENDOV cleavage position, samples were run on a 20% sequencing gel together with 32 P-labelled RNA oligonucleotides of defined lengths (13–16 nt; Supplementary Table S1 , primers 16–19). The results were visualized by phosphorimaging (Typhon 9410, Amersham Biosciences) and quantified with ImageQuant TL (Molecular Dynamics). Full size images of all panels presented are found in Supplementary Fig. S3 in the order they appear in the manuscript. For the single-turnover assays, 5 nM of endonuclease V was incubated with 1 nM substrate in 100-μl reaction volume using the same buffer as above. Samples were withdrawn after 3, 8, 15, 30, 60, 120, 300, 900, 1,800, 3,600 and 7,200 s and reactions stopped and analyzed as described above. Quenched samples were kept on ice until all time points were collected. Results were visualized and quantified as above. For the calculation of the catalytic turnover rate k obs (s −1 ), a one phase association model was fitted to three parallel data sets. Modelling A model of human ENDOV in complex with DNA dI rG was constructed by superposing the homology model of human ENDOV [21] with the T. maritima EndoV in complex with incised DNA [44] (PDB id 2W35 ) and subsequently replacing the dG 3′ to the inosine with an rG nt retrieved from a 0.95-Å resolution X-ray structure of a double-helix RNA fragment [45] (PDB id 3NJ6 ). Cell culture and Northern blot analysis Human epithelial glioblastoma cells U373-MG (American Type Culture Collection) were cultured in Dulbecco’s modified Eagle’s medium (Gibco) supplemented with 10% fetal calf serum (PAA lab), 1x GlutaMAX (200 mM, Gibco) and 1 × penicillin–streptomycin (Lonza) at 37 °C in 5% CO 2 atmosphere. Total tRNAs were isolated using RNAzol RT (Molecular Research Center) according to the manufacturer’s recommendations. Gel electrophoresis showed that the isolates contained mainly tRNA. Total tRNA (4.5 nM) was incubated with ENDOV (0.3 and 0.6 μM) as described under activity assays. After heat denaturation at 55 °C for 5 min, samples were separated by 15% PAGE in 1x taurine at 200 V for 50 min. The tRNA was transferred to a nylon membrane (Hybond XL, GE Healthcare) by electroblotting in 1x taurine at 4 °C, 5 V and over night. RNA was UV-crosslinked to the membranes (120 mJ cm −2 in a CL-1000 UV-Crosslinker, UVP). The Northern Max kit (Ambion, Applied Biosystems) was used for prehybridization, hybridization and washing steps as described by the manufacturer. 32 P 5′-end-labelled oligonucleotides (Eurofins; Supplementary Table S3 ) complementary to the 5′-ends of tRNA Ser (AGA), tRNA Leu (AAG), tRNA Arg (ACG), tRNA Asp (GTC), tRNA Glu (CTC) and tRNA Lys (CTT) were used as probes. Hybridization signals were analyzed by phosphorimaging and ImageQuant TL software. If endonuclease V incises the tRNA at the wobble I, the expected size of the 5′-cleavage product is 35 nt. Markers used were 32 P labelled RNA oligonucleotides (25 and 38 nt), which will migrate slightly faster than unlabelled fragments due to the negative charge of the phosphate label. Hybridized probes were removed from the filters by boiling in 0.1% SDS. Full size images of the Northern blots presented are found in Supplementary Fig. S3n–s . How to cite this article: Vik, E. S. et al. Endonuclease V cleaves at inosines in RNA. Nat. Commun. 4:2271 doi: 10.1038/ncomms3271 (2013).